Cooperative dual palladium/silver catalyst for direct difluoromethylation of aryl bromides and iodides Difluoromethylated arenes are one of the privileged structural motifs that are important for fine tuning the biological properties of drug molecules. No general catalytic method exists for the formation of difluoromethylarenes. Previous methods for the preparation of difluoromethylarenes typically required harsh conditions, multiple steps or stoichiometric amount of catalysts. Here we report a cooperative dual palladium/silver catalyst system for direct difluoromethylation of aryl bromides and iodides under mild conditions. We develop the system by initial preparation of the putative intermediates in the dual-catalytic cycles, followed by studying the elemental steps to demonstrate the viability of the proposed cooperative catalytic cycle. The reaction is compatible with a variety of functional groups such as ester, amide, protected phenoxide, protected ketone, cyclopropyl, bromide and heteroaryl subunits such as pyrrole, benzothiazole, carbazole or pyridine. It is a well-known fact that the incorporation of fluorine or fluoroalkyl groups into drug molecules will bring beneficial effects on the drug’s pharmacokinetic properties, binding selectivity and metabolic stability [1] , [2] . Consequently, the incorporation of fluorine or fluoroalkyl groups has become a daily routine in the design and fine tuning of the biological properties of the drug candidates. The difluoromethyl group (CF 2 H), like its analogue CF 3 group, has attracted increasing interests recently since the difluoromethyl group is known to be bioisostere of carbinol [3] , thiol [4] or hydroxamic acid hydroxyl group [5] . In addition, the difluoromethyl group can act as lipophilic hydrogen bond donor to improve the binding selectivity and cell membrane permeability. In sharp contrast to the numerous methods for trifluoromethylation of arene derivatives [6] , [7] , few methods for direct difluoromethylation of arenes under mild conditions have been reported [7] , [8] . Instead, difluoromethylarenes are typically accessed by deoxo gem -difluorination of the corresponding aldehydes with aminosulfurtrifluorides (DAST, Deoxofluor), BrF 3 ·Py or a combination of HF-pyridine and N -halo imide or amide [9] , [10] , [11] , [12] . Since these reactions were conducted under harsh reaction conditions and various functional groups were not compatible, many efforts have been made towards the development of alternative ways to introduce the difluoromethyl group into the desired position of the aromatic rings. Difluorination of benzylic C–H bonds that was promoted by visible light or silver catalyst generated difluoromethylarenes efficiently, yet selectivity is problematic for multi-alkylated arenes [13] , [14] , [15] . Baran and coworkers [16] , [17] reported a radical difluoromethylation of heteroarenes with zinc difluoromethanesulfinate, but reactions with arenes have not been reported. Several transition metal-catalysed difluoromethylation involved the using of difluoromethyl surrogates such as α-silyldifluoroacetate [18] and difluoromethylphenylketone [19] have emerged recently. Nevertheless, tedious protection/deprotection steps in these reactions significantly decreased the overall efficiency of the transformations. More recently, three copper-mediated direct difluoromethylation of aryl and vinyl iodides have been reported [20] , [21] , [22] . These transformations represent as a major step forward. However, the requirements of stoichiometric amount of copper salts, long reaction times or high temperatures limited their practical applications. In addition, the difluoromethylation of aryl bromides was not reported. Hence, new transition metal-catalysed method for direct difluoromethylation of aryl substrates with simple reagents under mild reaction conditions represents an unmet challenge and is urgently needed. Herein, we report the development of a Pd/Ag bimetallic catalyst system that cooperatively catalysed the direct difluoromethylation of a broad range of aryl bromides and iodides with readily available reagent TMSCF 2 H as the difluoromethyl source under mild conditions. The difluoromethylation method was compatible with a wild range of functional groups. The utility of this method is demonstrated by the efficient difluoromethylation of three drug-like candidates. The introduction of a difluoromethyl group into a molecule of interest at a late stage of a synthesis under mild reaction conditions could accelerate the discovery of a lead compound. Catalyst design Our design of a cooperative dual Pd/Ag bimetallic catalyst [23] , [24] , [25] , [26] , [27] , [28] for direct difluoromethylation of aryl halides was inspired by a classical cross-coupling reaction—Sonogashira reaction [29] . It was proposed that the palladium-catalysed alkynylation of aryl halides was catalysed by a two-component catalyst system consisting of two different transition metal complexes (Pd/Cu), in which the palladium-catalysed activation of aryl halides was cooperatively coupled through a transmetalation process with the catalytic route of in situ formation cuprous acetylides in the presence of an amine. We reasoned that if a similar cooperative bimetallic catalyst system could be created, in which aryl halide and the difluoromethyl reagent would be activated simultaneously in a substrate-selective manner by palladium and a second coinage metal catalyst, followed by cooperative transmetalation of the resulting two different active metallic species, and further reductive elimination from [L 2 Pd(Ar)(CF 2 H)] complex to produce the desired coupled product, a highly efficient and practical synthetic method for the introduction of the difluoromethyl group into arenes and heteroarenes could be developed ( Fig. 1 ). To create such a cooperative bimetallic catalyst system, we are immediately facing several challenges. First, difluoromethylated palladium complexes [L 2 Pd(Ar)(CF 2 H)] are unknown and reductive elimination from an Ar-Pd-CF 2 H complex, the key product-forming step, has never been observed; Second, difluoromethylated coinage transition metal species in low oxidation states are known to be thermally unstable [30] , [31] . Thus, a ligand that can stabilize the difluoromethylated complexes must be identified; Third, even if [L-M-CF 2 H] is stable enough, the transmetalation step that transfers the difluoromethyl group from [L-M-CF 2 H] to [L 2 Pd(Ar)(X)] must be substantially faster than the decomposition of [L-M-CF 2 H] in solution. Fourth, most importantly, the two operating catalytic cycles should be compatible. The reagents, ligands and the catalysts from both catalytic cycles should not interfere with each other to interrupt the catalytic reaction. 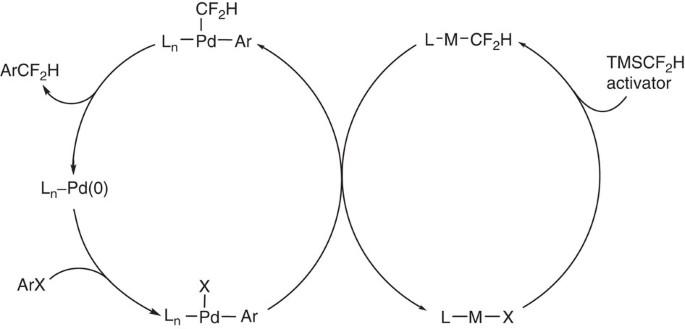Figure 1: Proposed cooperative bimetallic catalytic system for direct difluoromethylation of aryl halides. M, coinage metals such as Ag, Cu or Au; L and Ln, ligands; X, anionic ligands, such as chloride, bromide, iodides andtert-butoxide. Figure 1: Proposed cooperative bimetallic catalytic system for direct difluoromethylation of aryl halides. M, coinage metals such as Ag, Cu or Au; L and Ln, ligands; X, anionic ligands, such as chloride, bromide, iodides and tert -butoxide. Full size image Synthesis of [(DPPF)Pd(Ar)(CF 2 H)] complexes We started our investigation by the development of synthetic routes for the preparation of difluoromethylated palladium complexes [L 2 Pd(Ar)(CF 2 H] that will promote reductive elimination to form ArCF 2 H and a difluoromethylated coinage metal complex that is stable enough to transfer the difluoromethyl group to aryl palladium halide complex under the presumably required elevated reaction temperature ( Fig. 2 ). Initial attempts to synthesize [(DPPF)Pd(Ph)(CF 2 H)] by direct reaction of [(DPPF)Pd(Ph)(I)] with TMSCF 2 H in the presence of NaO t Bu, KO t Bu or CsF in various solvent such as THF, dioxane and toluene were unsuccessful. Instead, difluoromethane (CF 2 H 2 ) and tetrafluoroethane (HCF 2 CF 2 H), two self-decomposition side products from difluoromethyl trimethylsilane, were observed as the main products. We then developed an alternative approach for the formation of [(DPPF)Pd(Ar)(CF 2 H)] by first generation of [(TMEDA)Pd(Ar)(CF 2 H)], followed by ligand exchange reaction. Treatment of [(TMEDA)Pd(Ar)(I)] with 4.0 equivalents of TMSCF 2 H in the presence of 2.0 equivalents of NaO t Bu in THF at room temperature for 1.5 h formed the difluoromethylated complexes 2a – 2e in 47–83% yields. The TMEDA ligand could be easily exchanged by DPPF in THF to afford complexes 3a – 3e in 37–76% yields ( Fig. 2a ). The structure of complex 3c was unambiguously determined by single-crystal X-ray diffraction ( Fig. 2b ). 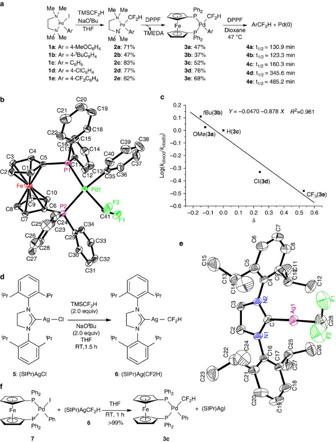Figure 2: Preparation of the putative intermediates and investigation of elemental reactions in the dual-catalytic cycles. (a) Formation of and reductive elimination from [(DPPF)Pd(Ar)(CF2H)].t1/2are the half-lives of the first-order reductive elimination kinetics. (b) X-ray structure of complex3c. ORTEP drawing at 50% probability; hydrogen atoms are omitted for clarity. (c) Hammett plot of rates of reductive elimination from (DPPF)-Pd(Ar-4-X)(CF2H) (3a–3e). (d) Formation of [(SIPr)Ag(CF2H)]. (e) X-ray structure of complex6. ORTEP drawing at 50% probability; hydrogen atoms are omitted for clarity. (f) Reaction of [(SIPr)Ag(CF2H)]6with [(DPPF)Pd(Ph)(I)]7. Figure 2: Preparation of the putative intermediates and investigation of elemental reactions in the dual-catalytic cycles. ( a ) Formation of and reductive elimination from [(DPPF)Pd(Ar)(CF 2 H)]. t 1/2 are the half-lives of the first-order reductive elimination kinetics. ( b ) X-ray structure of complex 3c . ORTEP drawing at 50% probability; hydrogen atoms are omitted for clarity. ( c ) Hammett plot of rates of reductive elimination from (DPPF)-Pd(Ar-4-X)(CF 2 H) ( 3a – 3e ). ( d ) Formation of [(SIPr)Ag(CF 2 H)]. ( e ) X-ray structure of complex 6 . ORTEP drawing at 50% probability; hydrogen atoms are omitted for clarity. ( f ) Reaction of [(SIPr)Ag(CF 2 H)] 6 with [(DPPF)Pd(Ph)(I)] 7 . Full size image Reductive elimination from [(DPPF)Pd(Ar)(CF 2 H)] complexes To assess the ability of complexes 3a – 3e to undergo reductive elimination, which is the key product-forming step in the catalytic cycle, we heated solutions of these complexes in dioxane at 47 °C. In the presence of 1.0 equivalent of dppf to trap the Pd 0 product, the difluoromethylated complexes 3a – 3e formed difluoromethylated arenes in 92–99% yields. Interestingly, these results indicated that the reductive elimination from a difluoromethyl palladium complex is much faster than those of its analogous CF 3 complex [32] , [33] , [34] , [35] . The rates of reductive elimination of difluoromethylarenes from complexes 3a – 3e at 47 °C were monitored by 19 F NMR spectroscopy. Reactions of these complexes were first order for greater than three half-lives. In addition, the rate of reductive elimination of 3b was independent of the concentration of DPPF. These results strongly suggest that reductive elimination occurs directly from these complexes. The rate constants for reductive elimination from complexes with electron-rich aryl groups were faster than those with electron-poor aryl groups. A good correlation was observed between Log( k obs / k obs(H) ) ( k obs(H) = k obs for 3c ) and Hammett parameters based on ionization of benzoic acid (σ) ( Fig. 2c ). The slower reductive elimination from complexes with more electron-withdrawing groups is likely due to ground-state effects such as stronger Pd–Ar bonds in these complexes. This argument has been used previously to rationalize the faster rate of reductive elimination from [(DPPF)Pt(C 6 H 4 -4-CF 3 )(C 6 H 4 -4-NMe 2 )] than from [(DPPF)Pt(C 6 H 4 -4-CF 3 )(C 6 H 4 -4-CF 3 )] (ref. 36 ). Synthesis of [(SIPr)Ag(CF 2 H)] complex We next turned our attention to identify a ligand to stabilize difluoromethylated coinage metal complexes. Because strong σ-donating N -heterocyclic carbenes (NHCs) have successfully been employed in stabilizing many coinage metal complexes [37] , [38] , [39] , [40] , [41] , [42] , we sought to determine if NHC ligands could stabilize AgCF 2 H that was known to undergo homolytic cleavage of Ag-C(CF 2 H) bond to form HCF 2 · and Ag(0) even at −50 °C. It was found that NHC-ligated difluoromethyl–silver complex [(SIPr)Ag(CF 2 H)] (SIPr: 1,3-bis(2,6-diisopropyl phenyl) imidazolin-2-ylidene) 6 could be prepared in 82% yield by the reaction of [(SIPr)AgCl] with 2.0 equivalents of TMSCF 2 H in THF at room temperature in the presence of 2.0 equivalents of NaO t Bu ( Fig. 2d ). Complex 6 was isolated as white crystalline solid and was characterized by 1 H, 13 C, and 19 F NMR spectroscopy and elemental analysis. The structural assignment was ambiguously further confirmed by single-crystal X-ray diffraction ( Fig. 2e ). Complex 6 is air stable and light insensitive in the solid state. Transmetalation from [(SIPr)Ag(CF 2 H)] to [(DPPF)Pd(Ar)(I)] Importantly, the isolation of the stable [(SIPr)Ag(CF 2 H)] 6 permitted us to study the transmetalation of the difluoromethyl group from [(SIPr)Ag(CF 2 H)] to [(DPPF)Pd(Ar)(I)], which is the key step in the cooperative bimetallic catalyst system. Addition of [(SIPr)Ag(CF 2 H)] to a solution of [(DPPF)Pd(Ph)(I)] in THF at room temperature led to quantitative formation of [(DPPF)Pd(Ph)(CF 2 H)] and [(SIPr)AgI] within 1 h. Heating of the reaction mixture at 80 °C for 1 h generated PhCF 2 H in 97% yield as determined by 19 F NMR) spectroscopy and gas chromatography–mass spectrometry ( Fig. 2f ). The fact that the two successive transmetalation reactions that involved Si-to-Ag and then Ag-to-Pd are much faster than a direct Si-to-Pd transfer indicate that the difluoromethyl silver complex could act as a transmetalation shuttle for the cooperative bimetallic catalytic system. Scope of Pd/Ag-catalysed difluoromethylation Having established the elemental steps of the both catalytic cycles and the key transmetalation step between the two systems, we set out to examine whether the dual-catalytic reaction could be realized. We first accessed the effect of the various combinations of palladium catalyst and [(SIPr)AgCl] on the reaction of 4-biphenyliodide and TMSCF 2 H using NaO t Bu as the activator. To our delight, after initial optimization of the reaction conditions, we obtained 4-difluoromethylbiphenyl ( 9a ) in 90% yield after 4 h at 80 °C in dioxane when 5 mol% Pd(dba) 2 , 10 mol% dppf and 20 mol% [(SIPr)AgCl] were used as the catalysts. The absence of the Pd catalyst shut down the production of the difluoromethylated arene completely. Ligand DPPF proved to be crucial for the reactivity of the catalyst. Reactions using other bidentate or monodentate phosphine ligands gave the difluoromethylated arene in 0–58% yields ( Supplementary Table 1 ). The silver catalyst played a critical role in transferring the difluoromethyl group. Without the silver catalyst, the yield of the reaction was less than 40% even with elevated reaction temperature (120 °C) and prolonged reaction time (20 h). In addition, reactions using other silver salts as the catalyst were much less effective ( Supplementary Table 2 ). It is important to note that NaO t Bu should be used as the activator since no product was observed when CsF or KF was used as activator. The cooperative bimetallic system was applied to difluoromethylation of a broad range of aryl iodides and aryl bromides ( Fig. 3 ). The difluoromethylated arenes were isolated, purified with silica-gel flash chromatography and characterized via NMR and high-resolution mass spectrometry. In general, substrates with electron-donating or electron-withdrawing groups were difluoromethylated in good yields. A number of functional groups are compatible with the reaction conditions. Aryl halides with ester, amide, protected phenoxide, protected ketone, cyclopropyl, bromide and fluoride afforded the products in 58–96% yield. In addition, aryl halides with heteroaryl subunit such as pyrrole, benzothiazole, carbazole or pyridine also provided the difluoromethylated products in good yields, despite the challenge nature of these substrates. Notably, when both bromide and iodide were presented in the substrate, the weaker carbon–iodine bond was selectively difluoromethylated. Furthermore, the current protocol was reliable and convenient for the preparation of difluoromethylated arenes not only on milligram scale but also for multigram synthesis. Reaction of 4-bromo-3-fluorobiphenyl with TMSCF 2 H on a 10-mmol scale gave 1.80 g of pure 9m in 81% yield. 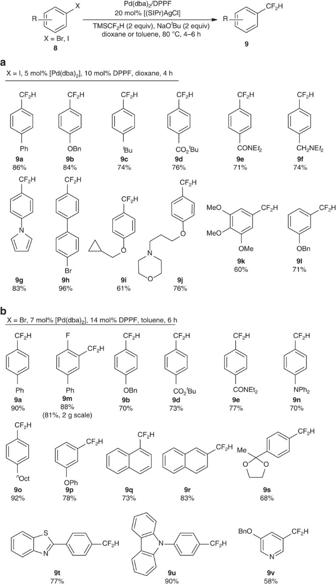Figure 3: Scope of the reaction. (a) Scope of cooperative bimetal-catalyzed difluoromethylation of aryl and heteroaryl iodides. (b) Scope of cooperative bimetal-catalysed difluoromethylation of aryl and heteroaryl bromides. Figure 3: Scope of the reaction. ( a ) Scope of cooperative bimetal-catalyzed difluoromethylation of aryl and heteroaryl iodides. ( b ) Scope of cooperative bimetal-catalysed difluoromethylation of aryl and heteroaryl bromides. Full size image As a demonstration of the synthetic applicability of the cooperative bimetallic catalyst, we studied the difluoromethylation of three medicinally important compounds. Compound 9w , a difluoromethylated analogue of a respiratory stimulant drug Etamivan used to treat chronic obstructive pulmonary disease [43] , was generated in 65% yield from its bromo-precursor. Likewise, compounds 9x and 9y , the difluoromethylation derivatives of nature hormone Estrone and antioxidant Vitamin E, occurred under the slightly modified bimetallic catalytic reaction conditions in 70 and 59% yields, respectively ( Fig. 4 ). These results suggest that the cooperative bimetallic catalyst system should be viable for the late-stage difluoromethylation of the leading compounds in drug discovery. 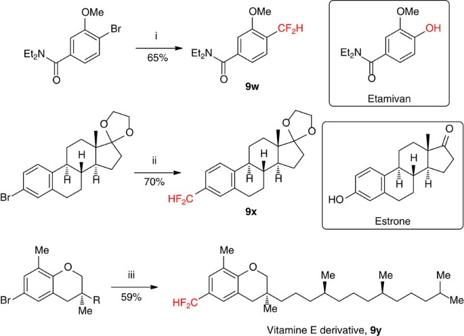Figure 4: Difluoromethylation of medicinally relevant compounds. Reactions were conducted on 0.5 mmol scale unless otherwise stated. Reported yields are for isolated materials. Reaction conditions: (i) 14 mol% Pd(dba)2, 28 mol% DPPF, 40 mol% [(SIPr)AgCl], 2.0 equiv. NaOtBu, 2.4 equiv. TMSCF2H, toluene, 80 °C, 6 h; (ii) 14 mol% Pd(dba)2, 28 mol% DPPF, 40 mol% [(SIPr)AgCl], 2.0 equiv. NaOtBu, 2.4 equiv. TMSCF2H, toluene, 80 °C, 48 h; (iii) 7 mol% Pd(dba)2, 14 mol% DPPF, 20 mol% [(SIPr)AgCl], 2.0 equiv. NaOtBu, 2.4 equiv. TMSCF2H, toluene, 80 °C, 48 h. Figure 4: Difluoromethylation of medicinally relevant compounds. Reactions were conducted on 0.5 mmol scale unless otherwise stated. Reported yields are for isolated materials. Reaction conditions: (i) 14 mol% Pd(dba) 2 , 28 mol% DPPF, 40 mol% [(SIPr)AgCl], 2.0 equiv. NaO t Bu, 2.4 equiv. TMSCF 2 H, toluene, 80 °C, 6 h; (ii) 14 mol% Pd(dba) 2 , 28 mol% DPPF, 40 mol% [(SIPr)AgCl], 2.0 equiv. NaO t Bu, 2.4 equiv. TMSCF 2 H, toluene, 80 °C, 48 h; (iii) 7 mol% Pd(dba) 2 , 14 mol% DPPF, 20 mol% [(SIPr)AgCl], 2.0 equiv. NaO t Bu, 2.4 equiv. TMSCF 2 H, toluene, 80 °C, 48 h. Full size image Because the bimetallic catalyst system involves two different catalytic cycles and many transition metal complexes, to probe the feasibility of the bimetallic catalyst system, it is essential to isolate and determine the structures of these intermediates and further study the elementary reactions of these complexes. Guided by the mechanistic assumption, we succeeded in the isolation of the key intermediates in the bimetallic catalyst system and proved the validity of the elementary steps, especially the transmetallation step between two catalytic cycles. On the basis of these solid mechanistic results, we developed a Pd/Ag bimetallic catalyst system that cooperatively catalysed the direct difluoromethylation of a broad range of aryl bromides and iodides with readily available reagent TMSCF 2 H as the difluoromethyl source under mild conditions. The difluoromethylation method was compatible with a wild range of functional groups. Considering the distinctive effects that fluoroalkyl group have on the properties of active pharmaceutical and agrichemical ingredients, the cooperative bimetallic catalyst system developed in this work provides a strategically new approach for the introduction of fluoroalkyl groups at the late stage of a medicinal chemistry development effort and may streamline the discovery of the lead compound. Nevertheless, further studies are clearly needed to understand the overall mechanism of the coupling process to improve the efficiency of the catalyst and to broad the scope the substrates such as aryl chlorides, vinyl halides and heteroaryl halides. General procedure In a Argon-filled glove box, ArBr or ArI (0.5 mmol, 1.0 equiv. ), Pd(dba) 2 (14.4 mg, 0.025 mmol, 0.05 equiv. ), DPPF (27.7 mg, 0.05 mmol, 0.1 equiv. ), [(SIPr)AgCl] (53.4 mg, 0.1 mmol, 0.2 equiv.) and NaO t Bu (96.1 mg, 1.0 mmol, 2.0 equiv.) were combined in a 20-ml vial. To this vial was added 5.0 ml of anhydrous toluene (dioxane for aryl iodides), followed by trimethyl(difluoromethyl)silane (148.8 mg, 1.2 mmol, 2.4 equiv.). The vial was sealed and moved out from the glove box. The mixture was stirred at 80 °C for 6 h (4 h for aryl iodides). The dark solution was diluted with H 2 O (15 ml). The mixture was filtered through a short plug of Celite, washed with CH 2 Cl 2 (20 ml × 3). The organic layer was combined, dried over NaSO 4 , filtered and concentrated under vacuum. The crude product was purified by column chromatography on silica gel with pentane/Et 2 O or pentane/EA mixture as the eluent to give the product. For NMR spectra of the compounds in this manuscript, see Supplementary Figures 1–108 . For general procedures and the procedure for the preparation of [(DPPF)Pd(Ar)(CF 2 H)] and [(SIPr)Ag(CF 2 H)], the procedure for reductive elimination from [(DPPF)Pd(Ar)(CF 2 H)] and transmetallation from [(SIPr)Ag(CF 2 H)] to [(DPPF)Pd(Ar)(I)], see Supplementary Methods . For the kinetic study of reductive elimination from complexes 3a – 3c , see Supplementary Methods . For representative decay of 3c as monitored by 19 F NMR spectra, see Supplementary Figure 109 . For the effect of the ligand on cooperative Pd/Ag-catalysed difluoromethylation, see Supplementary Table 1 . For the effect of different silver salts on cooperative Pd/Ag-catalysed difluoromethylation, see Supplementary Table 2 . Accession codes. The X-ray crystal structure information is available at the Cambridge Crystallographic Data Centre (CCDC) under deposition number CCDC 999362 and 975769 for the compound 2 and 6 reported in this communication. These data can be obtained free of charge from The Cambridge Crystallographic Data Centre via www.ccdc.cam.ac.uk/data_request/cif or pm application to CCDC, 12 Union Road, Cambridge CB2 1 EZ, UK [fax:+44-1223/336-033; deposit@ccdc.cam.ac.uk]. How to cite this article: Gu, Y. et al. Cooperative dual palladium/silver catalyst for direct difluoromethylation of aryl bromides and iodides. Nat. Commun. 5:5405 doi: 10.1038/ncomms6405 (2014).